A light-induced spin crossover actuated single-chain magnet Both spin-crossover complexes and molecular nanomagnets display bistable magnetic states, potentially behaving as elementary binary units for information storage. It is a challenge to introduce spin-crossover units into molecular nanomagnets to switch the bistable state of the nanomagnets through external stimuli-tuned spin crossover. Here we report an iron(II) spin-crossover unit and paramagnetic iron(III) ions that are incorporated into a well-isolated double-zigzag chain. The chain exhibits thermally induced reversible spin-crossover and light-induced excited spin-state trapping at the iron(II) sites. Single-chain magnet behaviour is actuated accompanying the synergy between light-induced excited spin-state trapping at the iron(II) sites and ferromagnetic interactions between the photoinduced high-spin iron(II) and low-spin iron(III) ions in the chain. The result provides a strategy to switch the bistable state of molecular nanomagnets using external stimuli such as light and heat, with the potential to erase and write information at a molecular level. It is a challenge to reduce the size of electronic devices and increase information density in materials area. As a result, molecules possessing magnetic bistable states are attracting a great deal of attention [1] , [2] , [3] , [4] , [5] , [6] , [7] , [8] , [9] , [10] , [11] , [12] , [13] , [14] , [15] , [16] , [17] , [18] , because these bistable states can act as elementary binary units (bits) used for information storage, providing potential applications in high-density information storage [3] , [5] , quantum computing [10] and spintronics [13] . In general, spin-crossover (SCO) complexes [1] , [2] , [3] , [4] , [5] , [6] , [7] and molecular nanomagnets [8] , [9] , [10] , [11] , [12] , [13] , [14] , [15] , [16] , [17] , [18] show such magnetic bistable states. SCO complexes show reversible transformation between a high-spin (HS) and a low-spin (LS) state [1] , [2] , [3] , [4] , [5] , [6] , [7] . In particular, the light-induced excited spin-state trapping (LIESST) [19] , [20] , [21] , [22] , [23] , [24] , [25] , [26] , [27] , [28] , [29] , [30] , [31] , [32] , [33] , [34] , which induces conversion of a LS state to a HS state by means of light irradiation, has attracted considerable interest. LIESST effects have been observed in various Fe II (or a few Fe III ) mononuclear complexes [19] , [20] , [21] , [22] , [23] , [24] . Moreover, SCO units and other paramagnetic ions have been linked via a short bridge to control intramolecular magnetic interactions [25] , [26] , [27] , [28] , [29] , [30] , [31] , [32] , [33] and generate magnetic ordering [34] via LIESST. However, no one has so far succeeded in introducing light-responsive SCO units into molecular nanomagnets, such as single-chain magnets (SCMs) and single-molecule magnets, to switch the bistable states of the nanomagnets. SCMs possess bistable states capable of interchanging between two magnetic polarization directions [14] , [15] , [16] , [17] , [18] . Although various types of SCMs have been synthesized, it is a challenge to produce and eliminate their bistable states using external stimuli, such as light, heat and so on [35] , [36] , [37] . The requirements for obtaining an SCM are uniaxial (Ising) anisotropy, strong intrachain magnetic interactions and weak interchain magnetic interactions [14] , [15] , [16] , [17] , [18] . Hence, the most effective approach towards tuning the SCM behaviour is to control directly the anisotropy of ions and intrachain magnetic interactions using external stimuli. LIESST can involve concomitant changes of spin state and anisotropy at the metal centres and subsequent changes of magnetic interaction pathways in the framework [19] , [20] , [21] , [22] , [23] , [24] , [25] , [26] , [27] , [28] , [29] , [30] , [31] , [32] , [33] , [34] . If the light-responsive SCO units can be incorporated in a chain, both the anisotropy of metal ions and the intrachain magnetic interactions will be tuned accompanying the LIESST effect [25] , [26] , [27] , [28] , [29] , [30] , [31] , [32] , [33] , [34] , producing a potential light-responsive SCM. Moreover, LIESST involves only one type of metal ion, providing the possibility to combine SCO units and various metal ions to produce photoswitchable SCMs. However, the LIESST effect has not yet been adopted successfully to switch the SCM behaviour. To synthesize a photoswitchable SCM using LIESST effect, the requirements of both SCM behaviours and LIESST effect should be considered. Until now, LIESST effects have been reported for Fe II and Fe III complexes [19] , [20] , [21] , [22] , [23] , [24] , [25] , [26] , [27] , [28] , [29] , [30] , [31] , [32] , [33] , [34] . Moreover, SCM behaviours have also been reported for complexes containing HS Fe II and LS Fe III ions [38] . Therefore, it is possible to obtain a photoswitchable SCM based on the LIESST effect of Fe II . Herein, we incorporate Fe II SCO units and paramagnetic LS Fe III ions into a cyanide-bridged {Fe III 2 Fe II } chain using the following building block: [Bu 4 N][Fe(Tp*)(CN) 3 ] (Tp*=hydrotris(3,5-dimethylpyrazolyl)borate). The cyanide bridges are supposed to link Fe II and Fe III ions into a chain and provide efficient superexchange pathways for strong magnetic interactions. The HS Fe II ion is paramagnetic (S=2) and usually has a strong anisotropy, whereas the LS Fe II ion is diamagnetic (S=0) and has no anisotropy, providing a switchable anisotropy. Moreover, the intrachain magnetic interactions between Fe III and Fe II ions can be switched accompanying the diamagnetic and paramagnetic transformations at the Fe II sites. The bulky Tp* ligand is introduced to avoid interchain magnetic interactions. Furthermore, a long ditopic, magnetically inert organic linker N,N′-bis-pyridin-4-ylmethylene hydrazine (bpmh) is adopted to tune the ligand field of Fe II sites, to provide the possible light-induced spin transition and to link the Ising chains into two-dimensional networks, maintaining a sufficiently large ratio of intra- to interchain magnetic interactions without changing the SCM behaviour significantly. Herein, based on the above strategy, the complex {[Fe III (Tp*)(CN) 3 ] 2 Fe II (bpmh)}·2H 2 O ( 1 ), composed of cyanide-bridged {Fe III 2 Fe II } chains, is synthesized. Complex 1 exhibits thermally induced reversible SCO and photoinduced spin transition at the Fe II sites. The SCM behaviour is switched, accompanying the synergy between the LIESST effect at the Fe II sites, and the ferromagnetic interactions between the photoinduced HS Fe II and LS Fe III ions in the chain. Structural characterization A crystal of the target compound was synthesized through reaction of complexes [Bu 4 N][Fe(Tp*)(CN) 3 ], bpmh and Fe(ClO 4 ) 2 ·6H 2 O in a methanol/water mixture placed in a test tube, using a diffusion method. Single-crystal X-ray diffraction analysis revealed that compound 1 crystallizes in a C 2/m space group ( Supplementary Table S1 and Supplementary Data 1 and 2 ). The crystal structure comprised layers of neutral mixed valence [Fe III (Tp*)(CN) 3 ] 2 Fe II (bpmh) and uncoordinated water molecules between them ( Fig. 1 and Supplementary Fig. S1 ). The layers were arranged in the ab plane and stacked along the c axis, and contained cyanide-bridged {Fe III 2 Fe II } double-zigzag chains running parallel to the crystallographic a axis ( Fig. 1a ). The Fe III 2 Fe II 2 square units exhibited two orientations of their mean planes, with a dihedral angle (hereafter denoted as φ ) between them. The chains were further linked by bis-monodentate bpmh ligands along the apical direction of the Fe II centres to a layer framework ( Fig. 1b ). The shortest interchain metal–metal distance was 10.69 Å. Such a large distance will minimize interchain magnetic interactions, providing the potential for an SCM behaviour without magnetic ordering. Within the neutral chain, each [Fe III Tp*(CN) 3 ] − entity linked two Fe II ions through two of its three cyanide groups in the cis positions, and each Fe II ion linked four [Fe III Tp*(CN) 3 ] − entities via coordination to cyanide nitrogen atoms, forming mixed-valence double-zigzag chains. The crystal structure contained one unique Fe III and one unique Fe II centre. The Fe III centre was coordinated to three nitrogen atoms from Tp* and three cyanide carbon atoms, and the Fe II centre was located in the elongated N 6 octahedral environment with four nitrogen atoms from CN − bridges and two nitrogen atoms from bpmh ligands. At 296 K ( Supplementary Table S2 ), the Fe II –N cyanide and Fe II –N bpmh distances were 2.158–2.162 and 2.179 Å, respectively, whereas the Fe III –C and Fe III –N bond distances were 1.893–1.926 and 1.976–2.020 Å, respectively. A comparison of these bond lengths with the reported examples suggested the Fe II centres to be Fe II HS , whereas the Fe III centre to be Fe III LS , forming Fe III LS (μ-CN)Fe II HS linkages [19] , [20] , [21] , [22] , [23] , [24] , [25] , [26] , [27] , [28] , [29] , [30] , [31] , [32] , [33] , [34] , [35] , [36] . The value of φ was 24.5°. 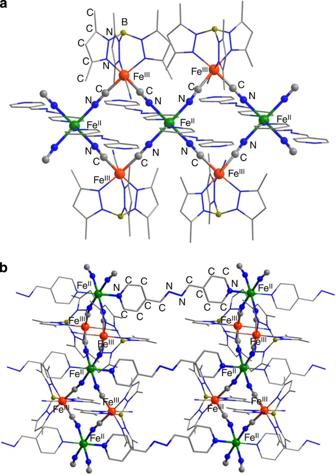Figure 1: Crystal structure of compound 1. The green, orange, grey, blue and dark yellow spheres represent FeII, FeIII, C, N and B atoms, respectively. Hydrogen atoms and solvent molecules have been omitted for clarity. (a) Structure of the chains. (b) Structure of the layers. Figure 1: Crystal structure of compound 1. The green, orange, grey, blue and dark yellow spheres represent Fe II , Fe III , C, N and B atoms, respectively. Hydrogen atoms and solvent molecules have been omitted for clarity. ( a ) Structure of the chains. ( b ) Structure of the layers. Full size image However, when crystals of compound 1 were cooled gradually to 13 K ( Supplementary Table S3 ), the Fe II –N bond distances were shortened by ~0.20 Å. At 13 K, the Fe II –N cyanide and Fe II –N bpmh distances decreased to 1.965−1.971 Å and 1.989 Å, respectively, which are characteristic of the LS Fe II ions [19] , [20] , [21] , [22] , [23] , [24] , [25] , [26] , [27] , [28] , [29] , [30] , [31] , [32] , [33] , [34] , [35] , [36] . The Fe III –C bond distances were 1.932–1.946 Å and the Fe III –N bonds distances were 1.987–2.020 Å, being nearly the same as those at 296 K. The value of φ was 22.8°. These temperature-dependent structural variations suggested that Fe II HS transformed to Fe II LS on cooling. Mössbauer spectra analysis The 57 Fe Mössbauer spectra were recorded at 300 and 5.0 K to characterize the electronic states of the Fe centres in compound 1 , to confirm the Fe II SCO ( Fig. 2 ). In the high-temperature phase at 300 K, one quadruple doublet was observed with Mössbauer parameters of δ (isomer shift)=0.04 mm s −1 and Δ E Q (quadruple splitting)=1.17 mm s −1 , which are characteristic of the LS Fe III species. Another quadruple doublet with a wide δ =0.60 mm s −1 and Δ E Q =1.66 mm s −1 showed the typical HS state of the Fe II species. The peak area ratio of the Fe II HS to Fe III LS species was 0.34/0.66, consistent with the results of the single-crystal analysis. When the temperature was cooled to 5.0 K, the quadruple doublet of Fe III , with δ =0.14 and Δ E Q =1.12 mm s −1 , remained nearly unchanged, whereas that of the Fe II HS species disappeared. Moreover, an additional doublet with δ =0.49 and Δ E Q =0.15 mm s −1 , corresponding to the Fe II LS species, was observed. The peak area ratio of the Fe II LS to the Fe III LS species was 1:2 at 5.0 K, suggesting that all Fe II HS species transformed to Fe II LS species during the transition from the high-temperature to the low-temperature phase. 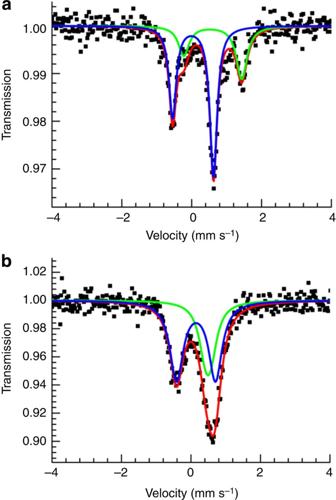Figure 2: Mössbauer spectra of compound 1. The solid lines represent Lorentzian curves plotted based on calculated values. (a)57Fe Mössbauer spectrum of compound1at 300 K. Mössbauer parameters:δ(isomer shift)=0.04 mm s−1and ΔEQ(quadruple splitting)=1.17 mm s−1, corresponding to the LS FeIII;δ=0.60 mm s−1and ΔEQ=1.66 mm s−1, corresponding to the HS FeII. (b)57Fe Mössbauer spectrum of compound1at 5.0 K. Mössbauer parameters;δ=0.14 mm s−1and ΔEQ=1.12 mm s−1, corresponding to the LS FeIII;δ=0.49 mm s−1and ΔEQ=0.15 mm s−1, corresponding to the LS FeII. Figure 2: Mössbauer spectra of compound 1. The solid lines represent Lorentzian curves plotted based on calculated values. ( a ) 57 Fe Mössbauer spectrum of compound 1 at 300 K. Mössbauer parameters: δ (isomer shift)=0.04 mm s −1 and Δ E Q (quadruple splitting)=1.17 mm s −1 , corresponding to the LS Fe III ; δ =0.60 mm s −1 and Δ E Q =1.66 mm s −1 , corresponding to the HS Fe II . ( b ) 57 Fe Mössbauer spectrum of compound 1 at 5.0 K. Mössbauer parameters; δ =0.14 mm s −1 and Δ E Q =1.12 mm s −1 , corresponding to the LS Fe III ; δ =0.49 mm s −1 and Δ E Q =0.15 mm s −1 , corresponding to the LS Fe II . Full size image Magnetic characterization Temperature dependence of the magnetic susceptibility ( χ ) of polycrystalline samples of compound 1 was measured between 1.8 and 300 K to better understand the spin transition. The χ T plot of the compound in cooling and heating modes under a magnetic field of 1,000 Oe is shown in Fig. 3a . At 300 K, the χ T product was 4.75 cm 3 mol −1 K, being typical for isolated metal ions of two LS Fe III ( S =1/2) and one HS Fe II ( S =2) in an octahedral coordination environment [38] . It was roughly constant down to 200 K. Lowering the temperature further, the χ T product decreased steeply from 4.75 cm 3 mol −1 K at 200 K to 1.21 cm 3 mol −1 K at 70 K, with an S -shaped curve being observed for SCO systems. On heating, the χ T value increased and returned to the initial value, without thermal hysteresis. The χ T product of 1.21 cm 3 mol −1 K corresponds to two isolated Fe III LS ions, suggesting that the Fe II HS ions were converted to the Fe II LS ions completely. Such results confirm a reversible SCO between the high-temperature phase with two Fe III LS ( S =1/2) and one Fe II HS ( S =2) metal ions and the low-temperature phase with two Fe III LS ( S =1/2) and one Fe II LS ( S =0) centres. The field-dependent magnetization at 1.8 K increased slowly to 1.95 Nβ at 50 kOe ( Fig. 3b ), indicating paramagnetic behaviours of the two isolated Fe III LS ions. Alternating current (ac) magnetic susceptibility was studied as a function of both temperature and frequency. No peaks and frequency dependence were observed for both in-phase ( χ ′) and out-of-phase ( χ ″) components ( Supplementary Fig. S2 ), which agrees with the paramagnetic behaviour of the low-temperature phase. 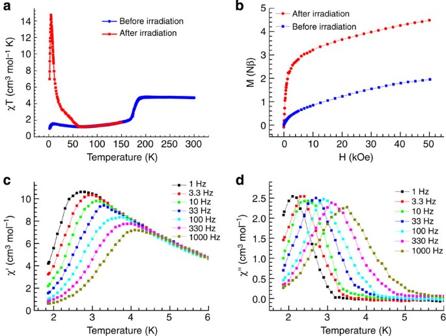Figure 3: Magnetic characteristics before and after light irradiation. Alternating current (ac) magnetic susceptibility characteristics after irradiation were performed in a zero dc field at various ac frequencies and with a 3.5 Oe ac field. (a) Temperature dependence susceptibilities of compound1before (blue squares) and after irradiation (red dots) in a dc field of 1,000 Oe. (b) Isothermal magnetization of compound1before (blue squares) and after irradiation (red dots) at 1.8 K. (c) Temperature dependence of the real parts of ac magnetic susceptibility after irradiation. (d) Temperature dependence of the imaginary parts of ac magnetic susceptibility after irradiation. Figure 3: Magnetic characteristics before and after light irradiation. Alternating current (ac) magnetic susceptibility characteristics after irradiation were performed in a zero dc field at various ac frequencies and with a 3.5 Oe ac field. ( a ) Temperature dependence susceptibilities of compound 1 before (blue squares) and after irradiation (red dots) in a dc field of 1,000 Oe. ( b ) Isothermal magnetization of compound 1 before (blue squares) and after irradiation (red dots) at 1.8 K. ( c ) Temperature dependence of the real parts of ac magnetic susceptibility after irradiation. ( d ) Temperature dependence of the imaginary parts of ac magnetic susceptibility after irradiation. Full size image Photomagnetic characterization On light irradiation (473 nm) at 5 K, a significant increase in the χ T values was observed because of the photoinduced spin transition from diamagnetic Fe II LS to metastable paramagnetic Fe II HS units ( Fig. 3a ). When the sample was heated from 2 K after irradiation, the χ T value increased steeply to a sharp maximum of 14.7 cm 3 mol −1 K at 4.6 K, which was much larger than the χ T value of 4.75 cm 3 mol −1 K measured at 300 K. The larger χ T value after irradiation suggested the presence of a magnetic interaction between the light-induced Fe II HS ( S =2) and the Fe III LS ( S =1/2) in the chain. The photoinduced magnetization relaxed to the initial value on a thermal treatment up to 62 K, indicating that the magnetization can be increased by irradiation with light and recovered with a thermal treatment ( Supplementary Fig. S3 ). After light irradiation, the field-dependent magnetization increased steeply below 10 kOe and then linearly to 4.49 Nβ for up to 50 kOe ( Fig. 3b ) on increasing the applied magnetic field, suggesting a ferromagnetic behaviour resulting from the ferromagnetic interactions between Fe III LS and photoinduced Fe II HS in the Fe III LS Fe II HS Fe III LS chain. The magnetization did not reach saturation even at 50 kOe, indicating the incomplete photoinduced spin transition and strong anisotropy of photoproduced Fe II HS . To investigate the magnetization dynamics after irradiation, ac magnetic susceptibility was studied as a function of both temperature and frequency. Variable-temperature ac susceptibility measurements revealed a strong frequency dependence of both χ ′ ( Fig. 3c ) and χ ″ ( Fig. 3d ), as was observed in case of other SCMs. The shift in the peak temperature ( T p ) is given by the parameter F =(Δ T p / T p )/Δ(log ω )=0.15, which lies in the expected range for an SCM, thus eliminating the possibility of a spin-glass behaviour. On the basis of these data, the relaxation times were estimated and fitted to Arrhenius laws ( Supplementary Fig. S4 ), providing a pre-exponential factor of τ 0 =5.0 × 10 −10 s and a relaxation energy barrier of Δ τ / k B =43.0 K. The value of τ 0 provides a quantitative estimation of the attempt time of relaxation from the chain bath and the obtained value is in good agreement with those reported for other SCMs [14] , [15] , [16] , [17] , [18] . In addition, harmonic analyses of the ac magnetic susceptibility (1 Hz) after irradiation ( Supplementary Fig. S5 ) showed that the ac signal does not contain χ 2 ω and χ 3 ω nonlinear magnetic susceptibility, suggesting that a single chain is magnetically isolated. A semicircular Cole–Cole diagram ( χ ″ versus χ ′, Supplementary Fig. S6 ) was constructed from the variable-frequency data collected at 2.5 K and fit to a generalized Debye model, yielding an α -value of 0.45. The α -value was large, indicating a broad distribution of the relaxation time, which may be due to the presence of defects in the chain, because unconverted LS Fe II atoms are present in the chain. This analysis demonstrates that compound 1 shows an SCM behaviour after irradiation. Relaxation of the photoinduced metastable state was monitored at different temperatures to probe the stability of the photoinduced phases ( Supplementary Fig. S7 ) [23] . In the high-temperature range (30–50 K), the relaxation time τ was strongly dependent on temperature because of the Arrhenius-type relaxation. In the low-temperature (5–10 K) region, relaxation time τ was less dependent on temperature, suggesting a temperature-independent tunnelling of the system from the metastable Fe III LS Fe II HS Fe III LS state to the stable Fe III LS Fe II LS Fe III LS state ( Supplementary Fig. S8 ). Density functional theory (DFT) calculations were carried out to estimate changes in electronic structures ( Fig. 4 and Supplementary Table S4 ). A three-cluster model was used to calculate the spin densities and electronic states of 1 ( Supplementary Tables S5 and S6 ). Supplementary Table S4 shows LS ferromagnetic (LSFM) state was the ground state and LS antiferromagnetic state was above 0.09 kcal mol −1 . DFT calculations indicate a weak ferromagnetic coupling between two Fe III LS ions. In the metastable HS state, HS ferromagnetic (HSFM) state was calculated to be 0.34 kcal mol −1 in the low-lying septet state. HS antiferromagnetic and HS ferro- and antiferromagnetic states were 3.14 kcal mol −1 in the triplet state and 2.16 kcal mol −1 in the quintet state, respectively. Thus, HSFM is also predominant in the metastable HS. These results suggest that a ferromagnetic exchange coupling between Fe III LS and Fe II HS units causes the predominant magnetic interaction in the double-zigzag chain in compound 1 . Calculated spin densities of three metal centres were Fe III LS (1.07), Fe II LS (0.08) and Fe III LS (1.05) in the LSFM state, and Fe III LS (1.09), Fe II HS (3.91) and Fe III LS (0.97) in the HSFM state ( Supplementary Table S4 ). 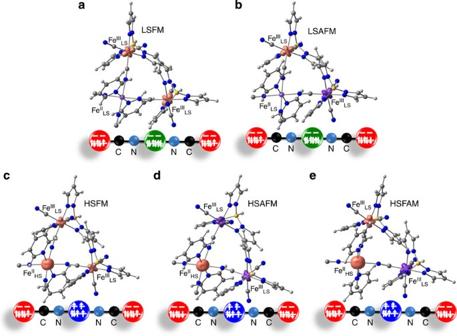Figure 4: Theα–βspin density of three cluster model. (a) LS ferromagnetic triplet state (LSFM), that is, FeIIILS(↑)–FeIILS–FeIIILS(↑). (b) LS antiferromagnetic singlet state (LSAF), that is, FeIIILS(↑)–FeIILS–FeIIILS(↓). (c) HS ferromagnetic septet state (HSFM), that is, FeIIILS(↑)–FeIIHS(↑↑↑↑)–FeIIILS(↑). (d) HS antiferromagnetic triplet state (HSAF), that is, FeIIILS(↓)–FeIIHS(↑↑↑↑)–FeIIILS(↓). (e) HS ferro- and antiferromagnetic quintet state (HSFAM), that is, FeIIILS(↑)–FeIIHS(↑↑↑↑)–FeIIILS(↓). Figure 4: The α – β spin density of three cluster model. ( a ) LS ferromagnetic triplet state (LSFM), that is, Fe III LS (↑)–Fe II LS –Fe III LS (↑). ( b ) LS antiferromagnetic singlet state (LSAF), that is, Fe III LS (↑)–Fe II LS –Fe III LS (↓). ( c ) HS ferromagnetic septet state (HSFM), that is, Fe III LS (↑)–Fe II HS (↑↑↑↑)–Fe III LS (↑). ( d ) HS antiferromagnetic triplet state (HSAF), that is, Fe III LS (↓)–Fe II HS (↑↑↑↑)–Fe III LS (↓). ( e ) HS ferro- and antiferromagnetic quintet state (HSFAM), that is, Fe III LS (↑)–Fe II HS (↑↑↑↑)–Fe III LS (↓). Full size image Furthermore, to support the occurrence of the LIESST effect, we measured the ultraviolet–visible–near infrared absorption spectra of the high-temperature phase, low-temperature phase and the low-temperature phase after photoirradiation ( Supplementary Fig. S9 ). When the HS state thermally changed to the LS state, the absorption peaks near 550 and 1,100 nm increased. This change in absorption intensity is induced by a spin transition from HS to LS at the Fe II sites, which has been confirmed via Mössbauer measurements and single crystal analysis. On the basis of previously reported results for Fe II SCO complexes, the broad absorption band near 550 nm for the low-temperature phase with Fe II LS can be mainly attributed to the metal-to-ligand charge transfer (MLCT) transition ( Supplementary Fig. S9 ). Furthermore, the absorption near 1,100 nm is probably attributable to the intervalence charge transfer from Fe II LS to Fe III LS . The photoinduced magnetization was observed when the compound was irradiated with 473 and 532 nm light; these wavelengths correspond to the excitation of the MLCT transition. When the LIESST effect is actually induced by light, the high-temperature phase should be generated. Indeed, when the complex with Fe II LS was irradiated at 8 K, the intensity of the peaks near 550 and 1,100 nm decreased. This result suggests that the low-temperature phase with Fe II LS transformed into the high-temperature phase with Fe II HS and is consistent with the occurrence of a spin transition because of light exposure. Notably, the photoinduced change is incomplete, because the interiors of the particles in the complex remain unchanged. To further confirm that the absorption change induced by light and temperature is consistent with the induction of a spin transition, time-dependent DFT calculations were used to calculate the excited-state energies, oscillator strengths and the electron density difference maps ( Supplementary Fig. S10 ). The time-dependent-DFT calculations show that the strong absorption near 550 nm is primarily because of the MLCT band. Similarly, the absorption near 1,100 nm for the low-temperature phase is because of the intervalence charge transfer from Fe II LS to Fe III LS . Thus, this result supports the conclusion that the thermally and photo-induced absorption changes are because of the spin transition in Fe II . In summary, Fe II SCO units and paramagnetic Fe III ions were alternated successfully in a double-zigzag chain. The SCM behaviour was switched with LIESST because of the formation of a ferromagnetic chain after irradiation. The present results provide an approach to combine the SCO and the SCM behaviour together to control the bistable state of molecular nanomagnets via LIESST effect, with the potential to erase and write information at a molecular level. Synthesis of compound 1 All reagents were available commercially and used without further purification. The compound [Bu 4 N][Fe(Tp*)(CN) 3 ] was synthesized according to a modified literature method [39] . A 1.0-ml aqueous solution containing 0.05 mmol of Fe(ClO 4 ) 2 ·6H 2 O was placed at the bottom of a test tube, and a 2.0-ml methanol solution containing 0.1 mmol of [Bu 4 N][Fe(Tp*)(CN) 3 ] and 0.1 mmol of bpmh was layered on the solution. Crystallization required several weeks, and crystals were obtained in 65% yield, based on Fe(ClO 4 ) 2 ·6H 2 O. The elemental analysis calculations yielded the following values for C 48 H 58 B 2 Fe 3 N 22 O 2 : C, 49.52; H, 5.02; and N, 26.47; on the other hand, the corresponding observed values were as follows: C, 49.56; H, 4.94; and N, 26.61. Mössbauer spectra measurements Mössbauer spectra (isomer shift versus metallic iron at room temperature) were measured using a Wissel MVT-1000 Mössbauer spectrometer with a 57 Co/Rh source in the transmission mode. Measurements at low temperature were performed using a closed-cycle helium refrigerator cryostat (Iwatani Co., Ltd). The sample was encapsulated in a sample holder to avoid loss of crystal water when pulling a vacuum on the cryostat. Ultraviolet–visible–near infrared spectroscopy Variable-temperature ultraviolet–visible–near infrared absorption spectra were measured using a UV-3100 (Shimadzu) with a helium-flow type refrigerator (Helitran LT-3-110). We measured the ultraviolet–visible–near infrared absorption spectra of the high-temperature phase, low-temperature phase and the low-temperature phase after photoirradiation. Thermogravimetric analysis Thermogravimetric analysis was performed at a rate of 10 °C min −1 under an Ar atmosphere using a TG/DTA Q600 system ( Supplementary Fig. S11 ). Magnetic studies Magnetic measurements of the samples were performed using a Quantum Design SQUID (MPMS-XL-7) magnetometer. On pumping at room temperature, the uncoordinated water molecules of compound 1 are removed easily, which may change the magnetic properties significantly. To prevent the loss of these uncoordinated water molecules, measurements were performed on finely ground microcrystalline powders of compound 1 restrained in a frozen eicosane matrix with polycarbonate capsules. Data were corrected for the diamagnetic contribution calculated from Pascal constants. Magnetic studies of the dehydrated samples were performed under a 1,000 Oe field in the temperature range from 2 to 400 K ( Supplementary Fig. S12 ). The sample was mounted into the SQUID machine and purged at 400 K to avoid the adsorption of water during the measurement. Photomagnetic measurements A powdered sample, which was spread on a commercial transparent adhesive tape, was used to study the photo-effects. The weight of the sample on the tape was determined by measuring the weight of the tape before and after spreading the sample and determining the difference. To prevent the loss of uncoordinated water molecules, the sample was introduced directly into the sample chamber at 100 K (He atmosphere) without purging. The photoirradiation of the samples was performed at 5 K with a laser diode pumped Nd:YAG laser ( λ =532 nm, 30 mW cm −2 , 12 h) or Nd:YAG laser ( λ =473 nm, 20 mW cm −2 , 12 h). The temperature-dependent magnetization was measured both before and after irradiation in the temperature range from 2 to 150 K. The difference in the magnetization before and after irradiation was extracted by subtracting the magnetization value before irradiation from that after irradiation. Furthermore, from these magnetization values and the sample weight, the difference in the χ T values before and after irradiation (Δ χ T) were calculated. Structure determinations and refinements The X-ray diffraction experiment for compound 1 was performed on a Rigaku charge-coupled device diffractometer using Mo-Kα radiation at 296 and 13 K. The structures were solved by a direct method and refined by full-matrix least-squares on F 2 using the SHELX programme with anisotropic thermal parameters for all non-hydrogen atoms. Hydrogen atoms were added geometrically and refined using the riding model. Computational methods A three-cluster model of compound 1 was optimized in the LS triplet state (LSFM) and the HS septet state (HSFM) using the DFT. After optimization, we carried out single-point calculations (for HS and LS) and obtained electronic structures of the LS antiferromagnetic, HS antiferromagnetic and HS ferro- and antiferromagnetic states. The B3LYP* function [40] was used. The SDD basis set [41] was used for Fe atom and the D95** basis set [42] for H, C, B and N atoms. The programme we used is Gaussian 09 (ref. 43 ). Accession codes: The X-ray crystallographic coordinates for structures reported in this study have been deposited at the Cambridge Crystallographic Data Centre (CCDC), under deposition numbers CCDC- 942943 (compound 1 at 296 K) and CCDC- 942942 (compound 1 at 13 K). These data can be obtained free of charge from The Cambridge Crystallographic Data Centre via www.ccdc.cam.ac.uk/data_request/cif . How to cite this article: Liu, T. et al. A light-induced spin crossover actuated single-chain magnet. Nat. Commun. 4:2826 doi: 10.1038/ncomms3826 (2013).